Superconductivity in the vicinity of antiferromagnetic order in CrAs One of the common features of unconventional superconducting systems such as the heavy-fermion, high transition-temperature cuprate and iron-pnictide superconductors is that the superconductivity emerges in the vicinity of long-range antiferromagnetically ordered state. In addition to doping charge carriers, the application of external pressure is an effective and clean approach to induce unconventional superconductivity near a magnetic quantum critical point. Here we report on the discovery of superconductivity on the verge of antiferromagnetic order in CrAs via the application of external pressure. Bulk superconductivity with T c ≈2 K emerges at the critical pressure P c ≈8 kbar, where the first-order antiferromagnetic transition at T N ≈265 K under ambient pressure is completely suppressed. The close proximity of superconductivity to an antiferromagnetic order suggests an unconventional pairing mechanism for CrAs. The present finding opens a new avenue for searching novel superconductors in the Cr and other transition metal-based systems. Transition-metal oxides or pnictides are rich in novel and intriguing electronic behaviours due to multiple quantum orders and competing phenomena. Among the different electronic states, the emergence of superconductivity in the vicinity of other quantum orders is at the heart of the exotic physics. Superconductivity has been observed in a majority of 3d transition-metal compounds except for the Cr- or Mn-based compounds in the sense that the low-lying states near Fermi level are dominated by their 3d electrons. It is thus of high interest to explore possible superconductivity in these systems. CrAs belongs to the large family of transition-metal pnictides with a general formula MX (M=transition metal, X=P, As, Sb), which form in either hexagonal NiAs-type ( B8 1 ) or orthorhombic MnP-type ( B31 ) structure (for review, see ref. 1 and references therein). At ambient conditions, CrAs adopts the MnP-type structure (inset of Fig. 1 ) with unit-cell parameters a =5.649 Å, b =3.463 Å and c =6.2084 Å. Its crystallographic and magnetic properties have been extensively investigated during 1970s due to the observation at T N =270±10 K of a first-order antiferromagnetic transition [1] , [2] , [3] , [4] , which is accompanied by discontinuous changes of lattice parameters. The most dramatic change is a sudden expansion of lattice constant b by ~4% below T N [5] . Neutron diffraction measurements established a double-helical magnetic structure propagating along the orthorhombic c axis with the Cr moment of 1.7 μ B lying essentially within the ab plane [3] , [4] . The acquisition of large Cr moment below T N has been rationalized as an itinerant to localized electron transition as a consequence of the sudden elongation of Cr-Cr separation along the b direction [2] . Previous studies have demonstrated a close relationship between the Cr magnetism and orthorhombic b axis length in the CrX series; with decrease in the size of X atom and thus the b axis, the Cr moment decreases from the full moment of 3 μ B per Cr for CrSb to 1.7 μ B per Cr for CrAs, and finally to nonmagnetic for CrP [1] . It seems that the magnetism of Cr in CrAs is located very close to the boundary of localized- to itinerant-electron transition. The coupled structural, magnetic and electronic degrees of freedom at T N in CrAs make external pressure a very effective knob in fine tuning its ground-state properties. Indeed, earlier high pressure studies have shown that the antiferromagnetic transition at T N can be readily suppressed by pressure and vanishes completely at P ~5 kbar (ref. 6 ). Since exotic phenomena such as the unconventional superconductivity are frequently observed in the vicinity of a magnetic quantum critical point, we are motivated to explore in great detail the physical properties of antiferromagnetic CrAs as T N is suppressed progressively under hydrostatic pressure. 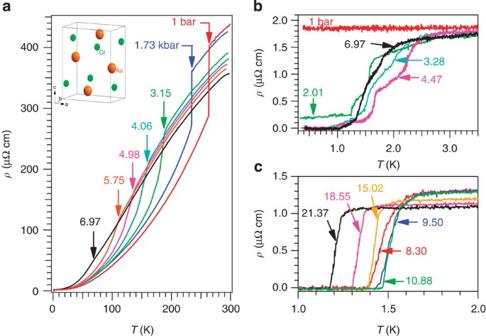Figure 1: High-pressure resistivity data. (a) Resistivityρ(T) of the CrAs single crystal under various hydrostatic pressures up toP=6.97 kbar in the whole temperature range highlighting the variation with pressure of the antiferromagnetic transition temperatureTNindicated by the arrows. (b,c)ρ(T) data at low temperatures in the whole investigated pressure range highlighting the evolution with pressure of the superconducting transition. The pressure values listed inaare the estimated pressure atTN, see Methods for details. The pressure values given inbandcare determined directly from the superconducting transition of Pb. A schematic crystal structure of orthorhombic MnP-type CrAs is displayed in the inset ofa. Figure 1: High-pressure resistivity data. ( a ) Resistivity ρ ( T ) of the CrAs single crystal under various hydrostatic pressures up to P =6.97 kbar in the whole temperature range highlighting the variation with pressure of the antiferromagnetic transition temperature T N indicated by the arrows. ( b,c ) ρ ( T ) data at low temperatures in the whole investigated pressure range highlighting the evolution with pressure of the superconducting transition. The pressure values listed in a are the estimated pressure at T N , see Methods for details. The pressure values given in b and c are determined directly from the superconducting transition of Pb. A schematic crystal structure of orthorhombic MnP-type CrAs is displayed in the inset of a . Full size image Here, we show that bulk superconductivity with T c ≈2 K emerges at the critical pressure P c ≈8 kbar, where the first-order antiferromagnetic transition at T N is completely suppressed. The close proximity of superconductivity to an antiferromagnetic order suggests an unconventional pairing mechanism for CrAs. As previous studies have shown that T N of CrAs can be suppressed by chemical substitutions at either Cr or As site [1] , our present work should open a new avenue for searching novel superconductors in the Cr and other transition metal-based systems. High-pressure resistivity We measured the resistivity ρ ( T ) of a number of CrAs single crystals under various hydrostatic pressures up to 21.4 kbar in a wide temperature range from 300 K down to 70 mK. The ρ ( T ) data of one represented sample shown in Fig. 1a illustrated the variation of T N with pressure (See the Methods section about how the pressure values at T N are estimated). As seen in Fig. 1a , the first-order antiferromagnetic transition is manifested as a sudden drop of resistivity at T N =264 K upon cooling at ambient pressure. As indicated by the arrows, T N decreases progressively with increasing pressure; the resistivity anomaly at T N changes from a sudden drop for P <3 kbar to a smoothly varied kink whose magnitude is also diminished gradually within the pressure range 3< P <7 kbar. Such an evolution of the resistivity anomaly at T N suggests a gradual crossover from strong to weak first-order transition, especially near the critical pressure where T N vanishes. It should be noted that in the previous high pressure study on a polycrystalline sample T N terminated at ~150 K under 5 kbar (ref. 6 ), whereas our measurements on a high-quality single-crystalline sample enabled us to track T N down to 70 K at P =6.97 kbar. Above this pressure, no anomaly can be discerned in resistivity at T >3 K. Our key finding of this study is the observation of superconductivity in CrAs with the application of high pressure. The ρ ( T ) data shown in Fig. 1b,c depict explicitly how the superconductivity emerges and then evolves with pressure at low temperatures. Below T N , ρ ( T ) measured outside the pressure cell does not show any anomaly down to 350 mK, thus confirming the absence of superconductivity in CrAs at ambient pressure. Interestingly, when the sample was subjected to a minute pressure <3 kbar, ρ ( T ) starts to decrease below ~2.5 K and displays multi-step drops before reaching a constant, non-zero value near 1 K. The amplitude of resistivity drop grows progressively with pressure, and eventually reaches zero resistivity near 1 K at P ≈3 kbar, signalling the occurrence of superconductivity. Upon further increasing the pressure in the range 3< P <7 kbar where T N remains finite, the superconducting transition is featured by similar multi-step drops; the onset temperature first increases and then decreases with pressure, while the zero-resistivity temperature T c 0 ≈1 K remains nearly constant. The multi-step feature fades away with further increasing pressure, and is finally changed to a single transition for P >8 kbar where T N vanishes completely. This indicated that the multi-step drop of resistivity at P <8 kbar should be caused by the two-phase coexistence as confirmed below by the AC magnetic susceptibility. As seen in Fig. 1c , T c 0 first increases and reaches a maximum of 1.47 K at P =10.88 kbar, above which it decreases gradually and reaches 1.17 K at 21.37 kbar, the maximum pressure of the present study. It should be noted that the pressure-induced superconductivity in CrAs, as well as the peculiar features of resistivity shown in Fig. 1 are well reproducible as confirmed on three independent CrAs single crystals with the residual resistivity ratio RRR>200. AC magnetic susceptibility The above resistivity results revealed that superconducting state coexists with the antiferromagnetically ordered state within a broad pressure range <7 kbar; the progressive development of the resistivity drop and the multi-step feature of superconductivity transition signal the growth of superconducting state at the expense of the antiferromagnetic state. To gain insights into the competing nature of these two states and to further verify the bulk nature of the observed superconductivity, we resorted to AC magnetic susceptibility measurements that can probe the diamagnetic signal due to superconducting transition. As shown in Fig. 2 , the diamagnetic signal starts to appear at P >3 kbar, and the superconducting shielding fraction grows steadily with pressure, reaching >90% of the sample volume at P >8 kbar. These results thus confirmed directly the bulk nature of pressure-induced superconductivity in CrAs. In addition, the onset temperatures of the diamagnetic signal are also in excellent agreement with the ρ ( T ) data shown in Fig. 1c . 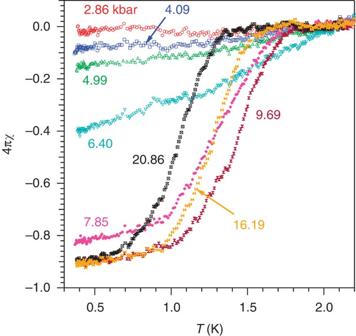Figure 2: AC magnetic susceptibility. Temperature dependence of the AC magnetic susceptibility 4πχof a CrAs single crystal under various hydrostatic pressures. The pressure values shown in the figure are determined directly from the superconducting transition of Pb. Figure 2: AC magnetic susceptibility. Temperature dependence of the AC magnetic susceptibility 4 πχ of a CrAs single crystal under various hydrostatic pressures. The pressure values shown in the figure are determined directly from the superconducting transition of Pb. Full size image Temperature–pressure phase diagram On the basis of the above results, we can construct a temperature–pressure phase diagram for CrAs single crystal. As seen in Fig. 3 , the first-order antiferromagnetic transition temperature T N =264 K at ambient pressure can be suppressed quickly by the application of external pressure; an extrapolation of T N ( P ) curve gives a critical pressure P c ≈8 kbar where T N approaches zero temperature. At P ≥ P c , bulk superconductivity with shielding fraction >90% is realized accompanied with an order of magnitude decrease of the 10–90% superconducting transition temperature width ΔT c , as seen in Fig. 3b . In this pressure region, the superconducting transition temperature T c exhibits a broad maximum at P ~11 kbar and then decreases gradually with further increasing pressure. For 3 kbar< P < P c , the superconducting state coexists with the antiferromagnetic state, and the volume fraction grows gradually at the expense of the other. It is interesting to note that the superconducting state in this pressure region is characterized by a higher onset temperature for superconductivity, Fig. 1b . 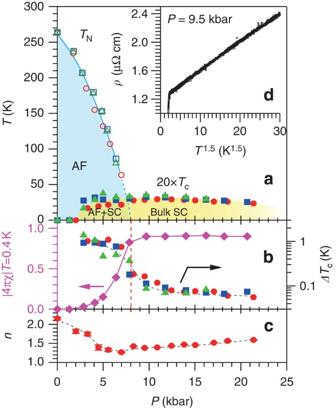Figure 3: Temperature–pressure phase diagram. (a) Pressure dependences of the antiferromagnetic (AF) transition temperatureTNand the superconducting (SC) transition temperatureTcfor CrAs single crystals;Tchas been scaled by a factor of 20 for clarity. (b) The superconducting shielding fraction at 0.4 K, |4πχ|T=0.4 K, and the superconducting transition temperature width,ΔTc, as a function of pressure. HereΔTcis defined as the 10–90% superconducting transition width. (c) Pressure dependence of the low-temperature resistivity exponent,n, obtained from the power-law fitting to the normal-state resistivity below 10 K. (d) A plot ofρversusT1.5for the normal-stateρ(T) curve atP=9.5 kbar. The symbols of circle (red), square (blue) and triangle (green) ina–crepresent three independent samples with residual resistivity ratio (RRR)=240, 327 and 250, respectively. Figure 3: Temperature–pressure phase diagram. ( a ) Pressure dependences of the antiferromagnetic (AF) transition temperature T N and the superconducting (SC) transition temperature T c for CrAs single crystals; T c has been scaled by a factor of 20 for clarity. ( b ) The superconducting shielding fraction at 0.4 K, |4 πχ | T =0.4 K , and the superconducting transition temperature width, ΔT c , as a function of pressure. Here ΔT c is defined as the 10–90% superconducting transition width. ( c ) Pressure dependence of the low-temperature resistivity exponent, n , obtained from the power-law fitting to the normal-state resistivity below 10 K. ( d ) A plot of ρ versus T 1.5 for the normal-state ρ ( T ) curve at P =9.5 kbar. The symbols of circle (red), square (blue) and triangle (green) in a – c represent three independent samples with residual resistivity ratio (RRR)=240, 327 and 250, respectively. Full size image The phase diagram of CrAs shown in Fig. 3a resembles that of many unconventional superconducting systems [7] , [8] , [9] , including the heavy-fermion, high- T c cuprate and iron-pnictide superconductors. As a universal trend in these systems, superconductivity emerges in the vicinity of a quantum critical point (QCP) where a high-temperature ordered state involving spin, charge or lattice degrees of freedom is suppressed via applying external tuning parameter δ , such as doping charge carrier, chemical or physical pressure. In addition, the superconducting transition temperature T c always passes through a maximum value at some critical δ c , leading to a dome-shaped T c - δ phase diagram. The proximity of superconductivity to a QCP lends strong support for the unconventional mechanism for Cooper pairing via the critical fluctuations. Despite the first-order nature of the antiferromagnetic transition in CrAs, the following observations suggested the presence of strong antiferromagnetic fluctuations near the critical pressure P c and the possible unconventional pairing mechanism. First, we found that within a large pressure regime of 3< P <21 kbar where superconductivity takes place, the normal-state ρ ( T ) <10 K follows the power-law relationship: ρ ( T )= ρ 0 + AT n with the exponent n falling in the range 1.5±0.1, as shown in Fig. 3c . This exponent is very close to the value predicated for incoherent scattering of quasiparticle via magnetic interactions in three-dimensional antiferromagnets [10] , [11] . One of the representative ρ ( T ) data at 9.5 kbar is plotted in the form of ρ versus T 1.5 in Fig. 3d . In our previous study [12] , we have shown that ρ ( T ) of CrAs single crystal at ambient pressure follows the Fermi liquid behaviour at T <10 K, with the Kadowaki–Woods ratio A / γ 2 falling onto the universal line of many correlated metals, where γ is the electronic specific heat coefficient. Our fitting to the ambient ρ ( T ) confirms the previous results with n =2.15(4). The observation of n <2 has been taken as a characteristic signature for non-Fermi liquid metals near a magnetic QCP [13] . Second, the antiferromagnetic fluctuations seem to be abundant above T N in that the magnetic susceptibility of CrAs keeps increasing with temperature up to at least 700 K under ambient pressure [12] . As a matter of fact, such an increasing behaviour of magnetic susceptibility has been found to be universal in the recently discovered iron-based superconductors, and regarded as an indication for antiferromagnetic fluctuations [9] . In this sense, these spin fluctuations would be optimized near the critical pressure where the antiferromagnetic order of CrAs is suppressed completely. Therefore, the critical spin fluctuations associated with the quantum criticality could act as an important glue medium for Cooper pairing. Last but not the least, the pressure-induced superconductivity in CrAs is found to be sensitive to the residual resistivity ρ 0 . Our initial high pressure studies on the CrAs crystals with ρ 0 ≈10 μΩ cm (residual resistivity ratio≈40–50) displayed indications of superconductivity at T <1 K, but no zero resistivity can be achieved. We finally confirmed the bulk superconductivity with higher T c on high-quality CrAs crystals having much reduced ρ 0 ≈1–2 μΩ cm. Such a sensitivity of superconductivity and the associated T c to disorders (impurities and/or defects) would imply an unconventional paring mechanism as found in the heavy-fermion superconductors [7] . In these cases, superconductivity is expected to be destroyed when the electron mean free path l mfp is smaller than the superconducting coherent length ξ . Our rough estimations of l mfp and ξ seem to verify such a scenario. We first estimated ξ near the optimal pressure from the upper critical field μ 0 H c2 , which is determined from the ρ ( T ) curves under different magnetic fields, Fig. 4a . 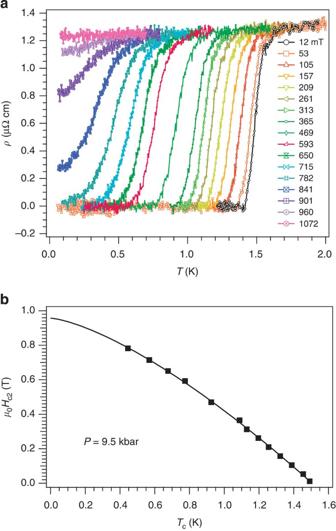Figure 4: Upper critical field. (a) Temperature dependence of resistivityρ(T) under different magnetic fields atP=9.5 kbar. HereTcvalues at different magnetic fields are determined as the middle point between 10 and 90% resistivity drop of the superconducting transition. (b) Temperature dependence of the upper critical fieldμ0Hc2for CrAs single crystal at 9.5 kbar. The solid line inbis a fitting curve with the empirical formula:μ0Hc2(T)=μ0Hc2(0) {1−[Tc/Tc(0)]α}, withμ0Hc2(0)=0.96(2) T,Tc(0)=1.506(6) K andα=1.41(6), respectively. Figure 4b displayed the μ 0 H c2 as a function of T c at P =9.5 kbar. Here, we determined T c as the middle point between 10 and 90% drop of resistivity. As shown in Fig. 4b , μ 0 H c2 versus T c can be fitted well with the empirical formula: μ 0 H c2 ( T )= μ 0 H c2 (0) {1−[ T c / T c (0)] α }, with μ 0 H c2 (0)=0.96(2) T, T c (0)=1.506(6) K and α =1.41(6), respectively. The obtained μ 0 H c2 (0) allows us to estimate the Ginzburg–Landau coherence length ξ =185 Å according to the relationship: μ 0 H c2 (0)= Φ 0 /2 πξ 2 , where Φ 0 =2.067 × 10 −15 Web is the magnetic flux quantum. On the basis of the measured Hall coefficient | R H |=2.6 × 10 −10 m 3 C −1 at 5 K, on the other hand, l mfp values of ~766 and 153 Å are obtained for the clean ( ρ 0 =2 μΩ cm) and dirty ( ρ 0 =10 μΩ cm) samples, respectively, by assuming a spherical Fermi surface with one kind of charge carrier. In spite of large uncertainty in the above estimations, we confirmed that bulk superconductivity can be seen only in samples with l mfp > ξ . Figure 4: Upper critical field. ( a ) Temperature dependence of resistivity ρ ( T ) under different magnetic fields at P =9.5 kbar. Here T c values at different magnetic fields are determined as the middle point between 10 and 90% resistivity drop of the superconducting transition. ( b ) Temperature dependence of the upper critical field μ 0 H c2 for CrAs single crystal at 9.5 kbar. The solid line in b is a fitting curve with the empirical formula: μ 0 H c2 ( T )= μ 0 H c2 (0) {1−[ T c / T c (0)] α }, with μ 0 H c2 (0)=0.96(2) T, T c (0)=1.506(6) K and α =1.41(6), respectively. Full size image Although superconductivity has been reported for some chromium alloys [14] , for example, Cr-Rh and Cr-Re, to the best of our knowledge, CrAs is the first superconductor among the Cr-based compounds. Unlike the alloys, most of the density of states near Fermi level for CrAs is attributed to the Cr-3d states [15] , which makes the magnetic degree of freedom relevant for the observed superconductivity. As a matter of fact, the itinerant-electron antiferromagnetism of chromium metal itself has been the subject of much interest for over 50 years [16] . To date, no unambiguous evidence of superconductivity has been observed near the QCP when the spin-density-wave antiferromagnetism of Cr is suppressed by either high pressure [17] , [18] or chemical doping [19] . In this regard, further theoretical and experimental studies are needed to elucidate the pairing symmetry and the dominant mechanism, especially the role of magnetism, for the observed superconductivity in CrAs. Sample preparation CrAs single crystals were grown out of the Sn flux. Details about the crystal growth procedures and sample characterizations at ambient pressure have been given elsewhere [12] . High pressure measurements High pressures were generated with a self-clamped piston-cylinder cell made of nonmagnetic BeCu and NiCrAl alloys [20] . Glycerol with a room temperature solidification pressure far >2 GPa was chosen as the pressure transmitting medium to minimize the shear stress when changing pressures at room temperature. The pressure ( P ) inside the piston-cylinder cell was monitored by detecting the superconducting transition temperature ( T c ) of a piece of Pb according to the equation: P (kbar)=( T 0 − T c )/0.0365, where T 0 =7.20 K is the T c of Pb at ambient pressure. It should be noted that the pressure inside the clamp-type pressure cell is not constant within the whole temperature range. It has been shown that the pressure drops ~3 kbar upon cooling down from room temperature to 4.2 K (ref. 21 ). Since the antiferromagnetic transition of CrAs spans over a large temperature range under pressures, we have to estimate the pressure at different temperatures properly. According to ref. 21 , the pressure is nearly constant below 90 K and it increases linearly to 300 K with a slope of 0.012 kbar K −1 for pressure <8 kbar. The pressure values at T N shown in Fig. 1a are estimated by the extrapolation: P ( T N )= P (Pb)+0.012 ( T N −90). The low temperatures down to 70 mK were reached by attaching the pressure cell to a Heliox-AC insert (Oxford Instrument) or dilution refrigerator. The resistivity was measured by the conventional four-probe method with the current applied along the orthorhombic a axis. AC magnetic susceptibility was measured with a mutual induction method at a fixed frequency of 317 Hz with a modulation field of ~2 Oe. The diamagnetic signal due to the superconductivity transition was estimated by comparing with the diamagnetic signal of Pb, which served as a pressure manometer, with nearly the same size as the CrAs sample. How to cite this article : Wu, W. et al . Superconductivity in the vicinity of antiferromagnetic order in CrAs. Nat. Commun. 5:5508 doi: 10.1038/ncomms6508 (2014).